Efficient power extraction in surface-emitting semiconductor lasers using graded photonic heterostructures Symmetric and antisymmetric band-edge modes exist in distributed feedback surface-emitting semiconductor lasers, with the dominant difference being the radiation loss. Devices generally operate on the low-loss antisymmetric modes, although the power extraction efficiency is low. Here we develop graded photonic heterostructures, which localize the symmetric mode in the device centre and confine the antisymmetric modes close to the laser facet. This modal spatial separation is combined with absorbing boundaries to increase the antisymmetric mode loss, and force device operation on the symmetric mode, with elevated radiation efficiency. Application of this concept to terahertz quantum cascade lasers leads to record-high peak-power surface emission (>100 mW) and differential efficiencies (230 mW A −1 ), together with low-divergence, single-lobed emission patterns, and is also applicable to continuous-wave operation. Such flexible tuning of the radiation loss using graded photonic heterostructures, with only a minimal influence on threshold current, is highly desirable for optimizing second-order distributed feedback lasers. Power extraction is a general and critical issue for the family of surface-emitting semiconductor lasers based on photonic crystal (PhC) resonators, be they 1D (second-order distributed feedback (DFB) lasers) [1] , [2] , [3] , [4] or 2D (surface-emitting PhC lasers) [5] , [6] , [7] , [8] , [9] , [10] , [11] . These devices operate on band-edge states of the photonic band structure, and can be classified as symmetric or antisymmetric, according to the spatial symmetry of their transverse electromagnetic field components. These two classes of modes have similar material and in-plane cavity losses, but exhibit significantly different radiation losses. Antisymmetric modes do not radiate in infinitely periodic structures, but become weakly radiative in finite-size devices, with low out-coupling efficiencies. In contrast, constructive interference generally occurs for symmetric modes; this leads to high radiation losses and highly efficient out-coupling [12] . Antisymmetric and symmetric modes are therefore usually termed non-radiative and radiative modes, respectively. Non-radiative modes are normally favoured in lasing owing to their lower total loss, but this leads not only to a limited extracted power (as discussed above), but also a far-field emission pattern that is double-lobed. Several strategies have been proposed to improve the power efficiency and beam patterns of second-order DFB lasers, including using gain-induced index depression in a DFB section [13] and chirped gratings [14] , [15] , [16] . However, these approaches are not as efficient or robust as desired. Nowadays, a commonly employed solution is the insertion of a central π -phase shift in devices operating on the fundamental non-radiative mode [1] , [17] , [18] , [19] . The field distribution becomes symmetric with respect to the centre of the device, but it remains antisymmetric within each unit cell of the grating. This solution enables a single-lobed beam pattern, but the power efficiency remains limited, as the field symmetry at the unit cell level is unchanged. An optimized design of grating and phase shift can lead to a uniform near-field distribution, which helps achieve single-mode emission over a large dynamic range, and gives (minor) improvements in power efficiency, as a uniform field distribution makes better use of the gain medium [17] , [18] . To address the drawback of operating on non-radiative modes, second-order DFB lasers operating on radiative modes using dual-slit gratings were recently reported [4] . However, the radiative mode still exhibits higher total loss than the non-radiative mode, and hence the operating spectral range and the output power improvement are constrained to a very small region around the laser peak gain. In this work, we demonstrate a novel concept to excite the fundamental radiative mode. A graded photonic heterostructure (GPH) is exploited to separate the field distribution of radiative and non-radiative modes spatially, by analogy with the spatial separation of electron and hole wavefunctions in a type-II semiconductor quantum well. Absorbing boundaries are implemented to increase the loss of the non-radiative mode selectively, and force the lasers to operate on a radiative mode with high power efficiency. We have applied this concept to second-order DFB terahertz frequency quantum cascade lasers (QCLs), where low power extraction remains a key issue and limits their widespread application [6] , [20] , [21] , [22] , [23] . Single-mode surface emission with record-high peak power and differential power efficiencies are demonstrated, as well as low-divergence single-lobed emission patterns and large operating spectral ranges. GPH resonators and absorbing boundaries In a 1D grating structure with uniform periodicity, radiative and non-radiative modes are located at the Γ -point of the photonic band structure. They have opposite curvatures and are separated by a photonic gap. 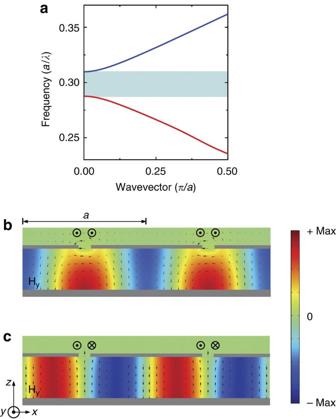Figure 1: Photonic band structure and mode distributions of a terahertz second-order DFB laser. A metal–metal waveguide structure is used, with the metallic grating formed directly on top of the active region. (a) Photonic band structure near the second band gap. A normalized frequency is used, whereais the periodicity of the grating. The blue horizontal band corresponds to the photonic band gap. (b,c) Transverse magnetic fields (Hy) of radiative and non-radiative band-edge modes (at the Γ-point of the band structure,kx=0), located above and below the band gap, respectively. The symbolsanddenote the direction ofHy. The arrows show the direction of the electric field. Their length is proportional to the amplitude of the electric field. Figure 1a shows the dispersion relation of these two bands in a terahertz DFB QCL based on metal–metal waveguides, and with the metallic grating formed directly on top of the active region (details of the specific terahertz QCL are given in Methods). The transverse magnetic fields ( H y ) of the two band-edge modes are plotted in Fig. 1b,c , respectively. The dispersion behaviours of the radiative and non-radiative bands are analogous to those of the conduction and valence bands in a semiconductor crystal; a uniform grating can thus be visualized as a bulk crystal. Borrowing the concept of type-II semiconductor quantum wells, where the wavefuctions of electrons and holes are separated, we can build a 1D GPH resonator. Photonic-band alignment aims to localize the radiative mode at the ridge centre, while pushing the non-radiative mode close to the laser facets. This spatial separation allows one to manipulate the material loss of each mode differently. An absorbing boundary condition is implemented, via a high-loss, n- doped layer located near the laser facets. The net effect is to increase the material loss of the non-radiative modes, without affecting the radiative ones. By correctly shaping the mode profile, a GPH thus permits selective excitation of the radiative mode and control of its radiative efficiency. Figure 1: Photonic band structure and mode distributions of a terahertz second-order DFB laser. A metal–metal waveguide structure is used, with the metallic grating formed directly on top of the active region. ( a ) Photonic band structure near the second band gap. A normalized frequency is used, where a is the periodicity of the grating. The blue horizontal band corresponds to the photonic band gap. ( b , c ) Transverse magnetic fields ( H y ) of radiative and non-radiative band-edge modes (at the Γ-point of the band structure, k x =0), located above and below the band gap, respectively. The symbols and denote the direction of H y . The arrows show the direction of the electric field. Their length is proportional to the amplitude of the electric field. 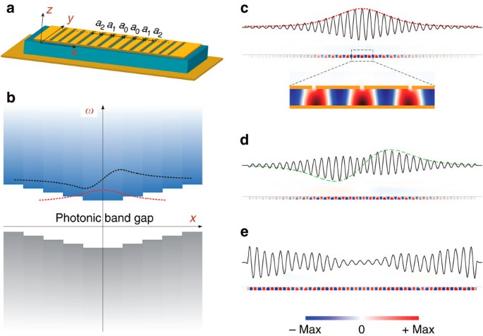Figure 2: The concept of GPH resonators. (a) Schematic illustration of a surface-emitting terahertz QCL with a GPH resonator. The top metallic grating is not periodic. Its lattice spacing (ai) is symmetrically and gradually decreased from the centre towards each end of the laser ridge, according to the recursive rule:ai+1=ai×0.99 (i=0, 1, 2, ...), whereaiis the periodicity ofi-th slit from the centre. In this work, the heterostructure contains 29 slits. (b) Schematic real-space photonic band diagram of the device. The vertical axis corresponds to the frequency of photons. The band structure is position-dependent, and smoothly shifts up in energy from the centre to each end of the device. Such a photonic band structure behaves simultaneously as a localizing potential for the radiative modes and as a barrier for the non-radiative modes. The red and black dotted curves are the schematic envelope functions of the first two confined radiative modes, respectively. The transverse magnetic field (Hy) along the cross-section of a device for the (c) first, and (d) second radiative modes, as well as the (e) first non-radiative mode are also illustrated. For each mode, the 1D sections ofHy, taken along a line through the centre of the active region, are also plotted as the black solid curves. For the two confined radiative modes, envelope functions, calculated using the envelope approximation, are also shown as the dashed curves in (c,d). Full size image Figure 2a shows a schematic diagram of a device with a GPH resonator. The top metallic grating is not periodic. Instead, its lattice spacing is symmetrically and gradually decreased from the centre towards each end of the laser ridge. As the band gap frequency scales with the periodicity in a PhC [24] , [25] , this structure features a position-dependent photonic band gap, which smoothly shifts upwards in energy from the centre to each end of the device. As a result, a V-shaped well for photons is formed, as shown in Fig. 2b . This configuration induces a localizing potential for the radiative modes: they are spatially trapped in the centre of the GPH resonator, and their frequency is quantized. In contrast, the same photonic potential behaves like a barrier for the non-radiative modes, which leak out of the grating region and experience large material losses from the highly doped GaAs contact layers, which are left in place at each end of the ridge. This judicious engineering of the GPH resonator therefore allows both selective excitation of the radiative mode—which is never the natural lasing mode in a photonic resonator—and engineering of the output power efficiency. Figure 2: The concept of GPH resonators. ( a ) Schematic illustration of a surface-emitting terahertz QCL with a GPH resonator. The top metallic grating is not periodic. Its lattice spacing ( a i ) is symmetrically and gradually decreased from the centre towards each end of the laser ridge, according to the recursive rule: a i +1 = a i ×0.99 ( i =0, 1, 2, ...), where a i is the periodicity of i -th slit from the centre. In this work, the heterostructure contains 29 slits. ( b ) Schematic real-space photonic band diagram of the device. The vertical axis corresponds to the frequency of photons. The band structure is position-dependent, and smoothly shifts up in energy from the centre to each end of the device. Such a photonic band structure behaves simultaneously as a localizing potential for the radiative modes and as a barrier for the non-radiative modes. The red and black dotted curves are the schematic envelope functions of the first two confined radiative modes, respectively. The transverse magnetic field ( H y ) along the cross-section of a device for the ( c ) first, and ( d ) second radiative modes, as well as the ( e ) first non-radiative mode are also illustrated. For each mode, the 1D sections of H y , taken along a line through the centre of the active region, are also plotted as the black solid curves. For the two confined radiative modes, envelope functions, calculated using the envelope approximation, are also shown as the dashed curves in ( c , d ). Full size image This qualitative analysis is supported by numerical simulations performed within a finite-difference time-domain (FDTD) approach [26] . Figure 2c,d,e shows the transverse magnetic field component ( H y ) along the cross-section of a device for the first two confined radiative modes, as well as the first delocalized non-radiative mode. The device parameters (see Fig. 2 ) correspond to the structures studied experimentally. Figure 2c shows that the fundamental radiative mode—whose transverse electromagnetic field is symmetric—is confined in the central part of the grating. The 1D sections of H y , taken along a line through the centre of the active region, are given for each mode (black solid curves). The quality ( Q ) factors of these three modes are 185, 128 and 52, respectively. Perfect metallic conductors are used in the FDTD simulation, with only the real part of the dielectric constant being used for the active region. The region close to the device facet, where the highly doped GaAs contact layer is left in place, is approximated as a perfectly absorbing boundary [6] . These Q -factors therefore reflect the total losses. The material losses induced by the metal (Au) and by the low-doped active region are not included, but they are the same for non-radiative and radiative modes. The result suggests that the first radiative mode will be the lasing mode, as it has a significantly higher Q -factor than the other two modes. It should be noted that the width of the grating slits is slightly modified to guarantee single-mode emission. As the radiation loss is also related to the effective emitting surface of the radiative modes, the slit width is increased in the region where the second radiative mode reaches its maximum. FDTD simulations show that such changes do not affect the spatial extension of the radiative/non-radiative modes. Instead, this selectively increases the radiation loss of the second radiative mode. This effectively enlarges the difference of the total loss between the first-order and the second-order radiative modes, and ensures the former is the lasing mode. Photonic heterostructures are non-periodic systems, which have typical dimensions significantly larger than the wavelength. Hence, a fully vectorial solution of Maxwell's equations represents a significant computational challenge. A simplified formalism, which is able to predict the relevant parameters of the GPH resonator, such as the frequency and spatial confinement of the modes, would be an extremely valuable tool. In particular, it would allow one to exploit fully the numerous degrees of freedom in the design. As highlighted in Fig. 2c,d , the magnetic field of the n -th photonic heterostructure mode can be expressed as the product of fast and slowly varying components, (ref. 27 ). H ( r ) is the unperturbed magnetic field of the related band-edge mode of the heterostructure constituent. It is a fast-varying field with periodicity equal to the lattice constant, but it is modulated by a slowly varying envelope function f n ( r ). The net power out-coupled by the device is determined by the extent of the envelope function f n ( r ) of the radiative mode, which satisfies a Schrödinger-like wave equation [28] , which in 1D is: Each heterostructure constituent is treated as a quasi-homogeneous medium described by an effective mass-like term, , which reflects the curvature of the local frequency dispersion at the Γ-point band edge; ω het ( x ) is the profile of the band-edge frequency in the GPH resonator; ω n is the eigenfrequency of the n -th mode in the GPH resonator. Once and ω het ( x ) are set, the eigenfrequency and envelope function of the modes can be immediately calculated using equation (1)—for instance with a simple transfer-matrix method—without returning to detailed electromagnetic simulations. Devices can then be designed using the envelope function approximation only. In this case, the normalized eigenfrequencies of the first two radiative modes are a 0 / λ =0.323 and 0.338, respectively, in good agreement with the results of fully vectorial FDTD simulations ( a 0 / λ =0.324 and 0.340, respectively). Here, a 0 is the periodicity of the slit at the centre of the photonic heterostructure. The bottom of the radiative band is a / λ =0.317, deduced from the 3D calculation of the photonic band. The related envelope functions, shown as dashed curves in Fig. 2c,d , are also in good qualitative agreement with the FDTD simulations. Performance comparison between GPH and DFB lasers Conventional second-order DFB lasers and lasers with GPH resonators (typical scanning electron microscope images of GPH lasers are shown in Fig. 3a ) were simultaneously fabricated on the same chip, using identical QCL material (wafer L421; see Methods) [29] . The DFB lasers are reference devices for performance comparison. Their grating duty cycle is 90%, to ensure uniform current injection, and the number of periods is 40—a trade-off between optimum total output power, slope efficiency and output-beam divergence. Ridge widths of 130 μm were used to obtain reasonable output power, and at the same time ensure operation on the fundamental transverse mode. For GPH lasers, the grating period decreases gradually from the centre to the end of the ridge, according to the recursive formula: ( i =0, 1, 2...), where a i is the periodicity of the i -th slit ( Fig. 2a ). The total number of periods of the GPH lasers is 29, which is already sufficient to confine the radiative mode. DFB lasers with different periodicities a , and GPH lasers with different a 0 , were fabricated to demonstrate on-chip frequency tunability. In both device architectures, absorbing boundaries are implemented by leaving in place (at the edges of the ridge resonators) highly doped GaAs contact layers uncovered by metal, as in refs 6 , 30 . 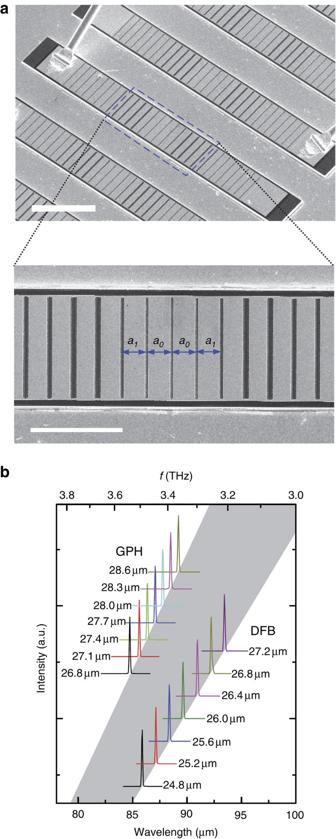Figure 3: Comparison of the spectra of GPH lasers with second-order DFB lasers. (a) Scanning electron microscope (SEM) images of GPH lasers with an expanded view of the GPH resonator. The scale bars in the upper and lower panels of the figure are 200 and 100 μm long, respectively. (b) Normalized emission spectra of GPH and second-order DFB lasers of different periodicities (afor DFB lasers anda0for GPH lasers, as marked in the figure). For clarity, each spectrum is shifted according to the periodicity. In both types of device, the emission wavelength tunes linearly with the periodicity (a/λ=0.29 for DFB anda0/λ=0.32 for GPH lasers). The grey region corresponds to the photonic band gap and highlights the fact that the GPH devices indeed operate on the higher-energy, radiative modes. Figure 3: Comparison of the spectra of GPH lasers with second-order DFB lasers. ( a ) Scanning electron microscope (SEM) images of GPH lasers with an expanded view of the GPH resonator. The scale bars in the upper and lower panels of the figure are 200 and 100 μm long, respectively. ( b ) Normalized emission spectra of GPH and second-order DFB lasers of different periodicities ( a for DFB lasers and a 0 for GPH lasers, as marked in the figure). For clarity, each spectrum is shifted according to the periodicity. In both types of device, the emission wavelength tunes linearly with the periodicity ( a / λ =0.29 for DFB and a 0 / λ =0.32 for GPH lasers). The grey region corresponds to the photonic band gap and highlights the fact that the GPH devices indeed operate on the higher-energy, radiative modes. Full size image Single-mode surface emission with a 30-dB side-mode suppression ratio was observed in all lasers, as shown in Fig. 3b (and also Fig. 4d,e ). The emission wavelengths scale linearly with the photonic lattice periodicity ( a for DFB, a 0 for GPH lasers), with normalized wavelengths a / λ =0.29 and a 0 / λ =0.32, respectively, in agreement with the simulations. Figure 3b demonstrates that the non-radiative mode in the DFB laser and the first radiative mode in the GPH lasers are active, separated by a frequency difference that corresponds to the photonic gap (the grey-highlighted region in Fig. 3b ). Lithographically controlled wavelength tuning ranges of 0.28 THz for DFB and 0.18 THz for GPH lasers are demonstrated. Larger tuning could be obtained by increasing the range of periodicities, as the tuning is only limited by the gain bandwidth of the active region. All of the DFB and GPH lasers operate in single mode at all the injected currents and for all the tested operation temperatures. This demonstrates unambiguously that the GPH concept is extremely robust, and well suited for use across a broad range of application sectors. 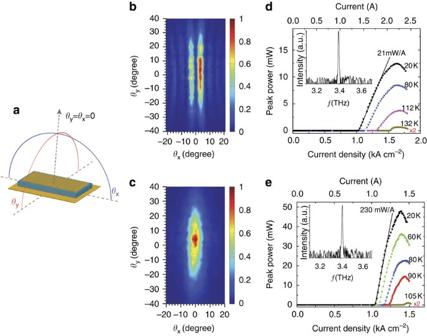Figure 4: Comparison of the far-field beam pattern and power extraction of GPH lasers with second-order DFB lasers. (a) Schematic diagram defining the scanning angles used in beam-profiling measurements. (b,c) The measured far-field patterns for typical second-order DFB and GPH lasers, respectively. The far-field emission of the GPH laser is naturally single-lobed, without introduction of phase shifts. (d,e) The light–current curves at different operation temperatures for a DFB and a GPH laser, respectively. Note, the two lasers have the same ridge width (130 μm) and exhibit the same emission wavelength, shown in the insets of (d,e), which is close to the active material peak gain. The GPH devices exhibit much higher power output and slope efficiency. Figure 4: Comparison of the far-field beam pattern and power extraction of GPH lasers with second-order DFB lasers. ( a ) Schematic diagram defining the scanning angles used in beam-profiling measurements. ( b , c ) The measured far-field patterns for typical second-order DFB and GPH lasers, respectively. The far-field emission of the GPH laser is naturally single-lobed, without introduction of phase shifts. ( d , e ) The light–current curves at different operation temperatures for a DFB and a GPH laser, respectively. Note, the two lasers have the same ridge width (130 μm) and exhibit the same emission wavelength, shown in the insets of ( d , e ), which is close to the active material peak gain. The GPH devices exhibit much higher power output and slope efficiency. Full size image Figure 4 shows the far-field emission patterns of the DFB and GPH lasers, respectively (measurement geometry shown in Fig. 4a ). Figure 4b shows that DFB lasers exhibit a double-lobed beam pattern with non-negligible side-lobe emission. In contrast, Fig. 4c demonstrates that GPH lasers have a purely single-lobed and focused beam pattern. Not only is this beneficial for use of terahertz QCLs in imaging and spectroscopy applications, but it also gives strong support to the premise that the GPH devices are operating on radiative modes, where the emission is naturally single lobed without any π -phase shift in the photonic lattice [31] , [32] , [33] . The most important aspect of this work, however, is that GPH lasers exhibit significantly higher power extraction and power slope efficiencies than DFB lasers. Figure 4d,e shows the light-current characteristics of typical devices operating at f =3.4 THz. The typical slope efficiencies and peak output powers of the DFB lasers at 20 K are 21 mW A −1 and 12 mW, respectively, comparable to the best reported results of second-order DFB lasers at similar wavelengths [2] , [4] . In contrast, the slope efficiency of the GPH lasers is 230 mW A −1 , more than one order of magnitude higher than their DFB counterparts. The FDTD simulations show that the radiation loss ( α rad ) is ~11 cm −1 for GPH lasers, and only ~0.5 cm −1 for DFB lasers. The significant improvement of slope efficiency is thus consistent with the theoretical calculations. At 20 K, the output power of the GPH lasers peaks at 50 mW, which is four times higher than that of the DFB lasers, despite the DFB lasers being almost 25% longer than the GPH structures. The different device lengths are the result of an endeavour to compare optimized GPH devices with optimized DFB lasers. If one fabricates DFB devices with the same length as the GPH structures, then the improved performance of GPH structures would be even more marked. The threshold current density ( J th ) of the GPH lasers is 1.08 kA cm −2 at 20 K, only slightly higher than that of DFB lasers (1.03 kA cm −2 ). Taking into account the material loss ( α mat ), which is of the order of 20–30 cm −1 for both kinds of lasers, the total loss ( α total ) of the GPH laser is approximately 30% larger than that of the DFB laser. The deviation in the differences between threshold current density and total loss is due to the fact that in terahertz QCLs based on the LO-phonon resonant depopulation mechanism, J th is mainly dominated by the strong parasitic current channel [34] , [35] . In fact, the total loss is best reflected by the maximum operation temperature ( T max ) of the lasers. As shown in Fig. 4d,e , the T max of GPH lasers (105 K) is lower than that of DFB lasers (132 K). We have increased the ridge width to 214 μm for GPH lasers fabricated from wafer L421. The devices still operate on the fundamental symmetric mode, with a significant improvement in laser performance. Supplementary Figure S1 shows the pulsed spectral and light-current characteristics of a typical wide-ridge GPH laser, as well as its far-field beam pattern. The GPH laser exhibits a record-high peak single-mode output power of 103 mW at 20 K—five times higher than the value obtained in terahertz DFB lasers with a dual-slit unit cell [4] , [36] . T max also increases up to 120 K and—extremely important for applications—the peak output power at liquid nitrogen temperatures is still 67 mW. The larger ridge resonator increases the surface area of light emission, and positions the lateral absorbing layers far away from the centre, hence reducing the material loss. This explains the higher T max . The full width at half maximum of the beam patterns are 9° and 20° in the directions along and perpendicular to the ridge axes, respectively. Continuous-wave (CW) operation of GPH lasers To demonstrate the CW operation of GPH lasers, we used a terahertz QCL based on a bound-to-continuum active region design (wafer V414; see Methods). This results in a lower applied bias and a lower threshold current density. The designed emission frequency was ~2.7 THz [37] . For lasers with bound-to-continuum active region, the parasitic current is less important and the threshold current density is mainly determined by the total waveguide loss. For this reason, GPHs were designed with shallower photonic wells and narrower slit widths to achieve a radiation loss of only α rad =7 cm −1 ; this is still, though, much larger than in the DFB counterpart ( α rad =0.5 cm −1 ). The total calculated waveguide loss of GPH lasers is thus about 20% higher than that of DFB lasers. 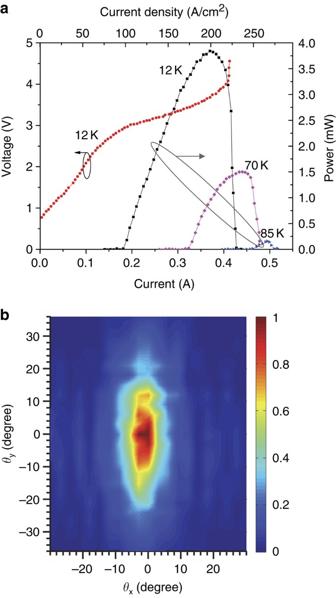Figure 5: GPH lasers operating in CW. (a) Light–current–voltage (L–I–V) curves of a typical GPH laser at different heat-sink temperatures. The ridge width is 127 μm, the ridge length is 1.46 mm and the single-mode emission frequency is 2.72 THz. (b) Far-field pattern of the same device measured at 78 K. Figure 5a shows the CW L–I–V curves of a typical GPH bound-to-continuum laser measured at different heat-sink temperatures: it operates CW up to 85 K, with a maximum output power of 3.8 mW and wall-plug efficiency of 0.3% at 12 K. This value of wall-plug efficiency is consistent with the current state-of-art. Figure 5b shows that this GPH laser also has an excellent, focused, single-lobed far-field beam pattern. For comparison, DFB lasers were also fabricated simultaneously on the same chip from the same wafer (see Supplementary Fig. S2 ). The GPH and DFB lasers had identical ridge widths and lengths, and very close emission frequency (~2.7 THz), which corresponds to the peak gain of the laser material. Figure 5 and Supplementary Fig. S2 demonstrate that the maximum output power of a GPH laser is six times higher than that from a DFB laser. At low temperature, J th of the GPH laser (100 A cm −2 ) is about 15% higher than that of the DFB laser (85 A cm −2 ), in qualitative agreement with the calculations of total losses. Furthermore, T max of the bound-to-continuum GPH laser is only 5 K lower than that of the DFB laser. In summary, GPH resonators can improve the power efficiency significantly, with only a minor influence on the device threshold current density and operation temperature. Figure 5: GPH lasers operating in CW. ( a ) Light–current–voltage ( L – I – V ) curves of a typical GPH laser at different heat-sink temperatures. The ridge width is 127 μm, the ridge length is 1.46 mm and the single-mode emission frequency is 2.72 THz. ( b ) Far-field pattern of the same device measured at 78 K. Full size image Further improvements in the CW output power can be achieved using GPH design, and utilizing higher-performing active region designs [38] . Another promising solution is to realize phase-locked arrays of GPH lasers [39] , from which much higher CW power and more directional emission is expected. We have demonstrated that it is possible to improve the output power in surface-emitting semiconductor lasers significantly by using GPH resonators and thereby engineering the material loss. This approach addresses the traditional-mode competition in second-order DFB lasers: the fundamental radiative modes can now be excited, yielding a very significant enhancement of slope efficiency and output power across a large spectral range, and at different heat sink temperatures. This is qualitatively different from previously reported solutions [4] , [12] , [13] , [14] , [15] , [16] , [17] , [18] , [19] . Furthermore, a very simple envelope-function approach allows one to design the GPH resonator by thinking in terms of photonic wells, without need for full electromagnetic simulations. The concept developed in this work can be exploited for dielectric grating DFB lasers, and the operation wavelength can also be extended to the mid- and near-infrared spectral ranges. When a dielectric grating is implemented on a semiconductor laser, light is generally preferentially emitted from the low-index component of the surface grating. For this reason, the symmetric mode always couples into the free space with a high radiation efficiency, whereas the antisymmetric mode does not. The photonic band structure of 1D grating is similar for both metallic and dielectric gratings, and the photonic band gap can be tuned by the index contrast. Especially, in the vast family of second-order DFB semiconductor lasers, the radiation loss is one or two orders of magnitude lower than the total loss. There is a large margin of design using a GPH resonator to greatly increase the power efficiency, with only a minor influence on the threshold current density and maximum operation temperature. Finally, this concept can be used in combination with quantum well or quantum cascade infrared photodetectors. Improvement of the surface coupling efficiency can be obtained, with the additional benefit of spatially concentrating the electromagnetic field in the detector cavity [40] , which is crucial to reduce the dark current. Modelling The photonic band structures of standard second-order DFB lasers were calculated by solving the 3D Helmholtz equation with Bloch periodic boundary conditions, using the commercial software Comsol Multiphysics. The quality factors of DFB and GPH lasers with finite ridge length were calculated by FDTD simulations, using the freely available package MEEP [26] . We performed two-dimensional FDTD simulations, considering an infinitely wide waveguide with absorbing boundary conditions. The metallization layers are considered to be perfect conductors, and only the real part of the refractive index of the semiconductor active region is taken into account. This approximation neglects the material loss caused by the metal and the low-doped semiconductor active region. Device fabrication The QCL structure (wafer L421) was grown by molecular beam epitaxy on an undoped GaAs substrate. After a 500-nm-thick undoped GaAs buffer layer, a 300-nm-thick Al 0.5 Ga 0.5 As etch-stop layer was grown, followed by a 75-nm-thick layer of GaAs n -doped with silicon at 5×10 18 cm −3 . The core consists of 226 stages of the active region, giving a total thickness of ≈10 μm. The design of the active region is based on a four-well structure with a longitudinal optical phonon resonant depopulation mechanism [41] . The growth was concluded by a 50-nm-thick GaAs capping layer, n -doped at 5×10 18 cm −3 . The growth parameters are similar for wafer V414, except that the active region is based on a bound-to-continuum design and its thickness is 12 μm. After growth, the QCL wafers were thermo-compressively bonded with gold onto a GaAs wafer following the procedure in ref. 42 , and the undoped substrates then removed by lapping and selective etching. The Al 0.5 Ga 0.5 As stop layers were selectively etched except in the regions where the wire-bonding pads are subsequently realized. The gratings and the wire-bonding pads were defined by contact optical lithography followed by metal deposition (Ti/Au, 8/400 nm) and lift-off. The doped GaAs contact layers in the grating slits were next removed by wet etching. Laser ridges were defined by inductively coupled plasma reactive ion etching. The top doped GaAs contact layer was left in place at each end of the ridges (50 μm in length) and also along the sides of the grating (5 μm in width) to provide absorbing boundary conditions. After polishing and back-contact deposition, the laser chips were cleaved and indium-soldered onto copper mounts for characterization in a continuous-flow helium cryostat. Measurement details The spectra, light–current ( L–I ) and current–voltage ( I–V ) characteristics were measured in pulsed mode (typically 0.3% duty-cycle, 500-ns-long pulses) for the devices fabricated from wafer L421, and in CW for devices fabricated from wafer V414. The spectral characteristics were measured using a Fourier transform infrared spectrometer (Bruker IFS66). The emitted power was measured by a calibrated DTGS photodetector and by a Thomas Keating absolute terahertz power-meter. The far-field emission patterns of the lasers were measured at 78 K with a Golay cell detector, which was scanned on a 15-cm-radius sphere centred on the device surface. The θ x = θ y =0 angle corresponds to the direction orthogonal to the device surface. How to cite this article: Xu, G. et al . Efficient power extraction in surface-emitting semiconductor lasers using graded photonic heterostructures. Nat. Commun. 3:952 doi: 10.1038/ncomms1938 (2012).